Carbon dioxide capture and conversion by an acid-base resistant metal-organic framework Considering the rapid increase of CO 2 emission, especially from power plants, there is a constant need for materials which can effectively eliminate post-combustion CO 2 (the main component: CO 2 /N 2 = 15/85). Here, we show the design and synthesis of a Cu(II) metal-organic framework ( FJI-H14 ) with a high density of active sites, which displays unusual acid and base stability and high volumetric uptake (171 cm 3 cm −3 ) of CO 2 under ambient conditions (298 K, 1 atm), making it a potential adsorbing agent for post-combustion CO 2 . Moreover, CO 2 from simulated post-combustion flue gas can be smoothly converted into corresponding cyclic carbonates by the FJI-H14 catalyst. Such high CO 2 adsorption capacity and moderate catalytic activity may result from the synergistic effect of multiple active sites. Due to the dependence on fossil fuels to meet the world’s growing energy demand, the concentration of CO 2 in the atmosphere has increased from 310 p.p.m. to over 380 p.p.m. during the last half century, and it continues to rise [1] , [2] , [3] . Some 60% of the total CO 2 emission worldwide is attributable to electricity generation [4] . The installation of effective CO 2 capture systems that can selectively remove the CO 2 component of the exhaust gas emitted by coal- or gas-fired power plants would extremely reduce the global annual emissions. Current technologies involving aqueous amine absorbents for the capture of CO 2 from a gas mixture are usually themselves significant consumers of energy and a source of corrosion problems in equipment [5] , [6] , [7] . Thus, exploration of new materials that can selectively and efficiently eliminate combustion-generated CO 2 is urgent. Due to their large capacity for the adsorption of gases and their chemical tunability [8] , [9] , [10] , [11] , [12] , [13] , [14] , [15] , [16] , [17] , [18] , [19] , [20] , [21] , the emerging porous metal-organic frameworks (MOFs) could serve as promising cost-effective and efficient materials for CO 2 capture and separation, but development of practically useful MOF materials for CO 2 capture directly from power plants remains a challenge. The flue gas generated from coal-fired power plant, released at a total pressure of approximately 1 atm., contains 15–16% CO 2 , 73–77% N 2 , 5–7% H 2 O, 3–4% O 2 and a small amount of acid gas [22] , [23] , [24] . An ideal MOF material for CO 2 capture should exhibit extraordinarily high CO 2 uptake and selectivity at ambient pressures; furthermore, it should also be resistant to water and acid gas, can be prepared on a large scale and is reusable. Moreover, in terms of practical applications, high volumetric CO 2 adsorption capacity seems even more important than gravimetric CO 2 adsorption capacity, since the capture and separation of post-combustion CO 2 is often carried out in a fixed-bed reactor [5] . Generally, open metal sites (OMS) and Lewis basic sites (LBS) are favorable for interaction with CO 2 and various types of OMS and LBS have been introduced into MOFs in an effort to improve their adsorption capacity [25] , [26] , [27] , [28] , [29] , [30] , [31] , [32] . To adsorb CO 2 effectively under ambient conditions, one would seek to prepare an MOF with high densities of OMS and LBS, in which the OMS and LBS could synergistically capture CO 2 molecules in the pores. Such a potential synergy effect from the OMS and LBS can improve the adsorption capacity more effectively than a single OMS or LBS. In this paper, we describe the design and synthesis of a Cu(II)-MOF, FJI-H14 with a high density of OMS and LBS, which shows extraordinary high volumetric uptake of CO 2 at ambient conditions and excellent selectivity for CO 2 over N 2 . Remarkably, it is highly stable in a water and acid/base environment and can be reused without loss of adsorption capacity; furthermore, it can be easily synthesized in large quantities. Experiments with simulated post-combustion flue gas have shown that FJI-H14 can smoothly catalyze the chemical transformation of CO 2 into the corresponding cyclic carbonates. Synthesis and structure analysis The reaction of 2,5-di(1 H -1,2,4-triazol-1-yl)terephthalic acid (H 2 BTTA, Fig. 1a ) with Cu(NO 3 ) 2 in H 2 O at 120 °C for 3 days affords rod-shaped blue crystals of FJI-H14 ([Cu(BTTA)H 2 O] n ·6nH 2 O) in 73% yield. 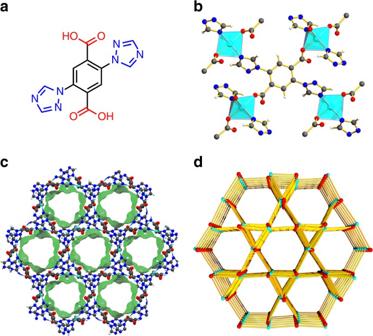Fig. 1 Structural illustration of FJI-H14.aThe selected ligand H2BTTA for the construction ofFJI-H14.bThe coordination environment of the Cu(II) ions as four-connected nodes and BTTA also as a four-connected node.cThe one-dimensional nanoporous channels along the crystallographiccdirection.dThe framework ofUSFtopology. (Cu atom, cyan; C atom, gray; O atom, red; N atom, blue; H atom, white) Single-crystal X-ray structure analysis shows that FJI-H14 crystallizes in trigonal space group R -3 (for more details see Supplementary Table 1 ). The crystallographic asymmetric unit contains one BTTA 2− ligand, one Cu(II) ion and one coordinate water. As shown in Fig. 1b , each Cu(II) ion has a square-pyramidal coordination geometry, and is surrounded by two imine N atoms from two different 1,2,4-triazole groups and two O atoms from two different carboxylate groups in the equatorial plane, together with one O atom of the water molecule in the vertex (Supplementary Fig. 1 ). Topologically, the Cu(II) ion is a planar 4-connected node, further linked by four tetradentate BTTA 2− ligands into a three-dimensional network with Kagome-like USF topology (Fig. 1d ). Consequently, there are hexagonal one-dimensional channels along the c direction (Fig. 1c ). The pore limiting diameter and the maximum pore diameter predicted by the program Poreblazer [33] for the fully evacuated FJI-H14 are 5.95 and 7.62 Å, respectively. 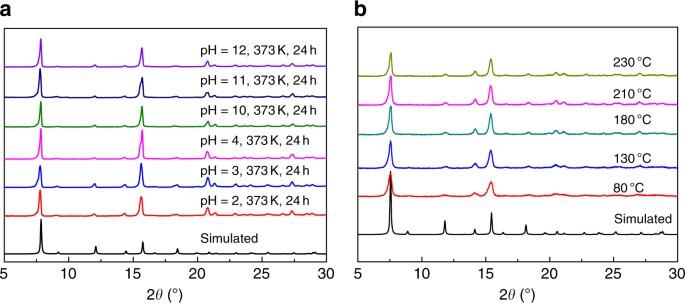Fig. 2 Stability of FJI-H14.aPXRD patterns after treatment with boiling water, acid/base environment from pH = 2 to 12 at 373 K.bTemperature-dependent PXRD patterns The evacuated FJI-H14 has a theoretical porosity of 44.4% according to PLATON calculations with a probe radius of 1.65 Å. FJI-H14 has a total concentration of active sites as high as 9.22 mol l −1 (the total of Cu(II) OMS is 3.07 mol l −1 and free N LBS is 6.15 mol l −1 ), which is higher than in many well-known MOFs for CO 2 capture (Supplementary Table 2 ). Fig. 1 Structural illustration of FJI-H14. a The selected ligand H 2 BTTA for the construction of FJI-H14 . b The coordination environment of the Cu(II) ions as four-connected nodes and BTTA also as a four-connected node. c The one-dimensional nanoporous channels along the crystallographic c direction. d The framework of USF topology. (Cu atom, cyan; C atom, gray; O atom, red; N atom, blue; H atom, white) Full size image Stability The flue gas from power plants contains moisture and acid gas, suggesting that the practical adsorbents of post-combustion CO 2 should be sufficiently stable toward heat, water and acid. This led us to investigate both the chemical stability and thermal stability of FJI-H14 before the CO 2 adsorption test. Powder X-ray diffraction pattern (PXRD) analyses reveal that FJI-H14 is very stable not only in boiling water but also in both acid and base environments at pH = 2 to pH = 12 and at temperatures as high as 373 K (Fig. 2a ). However, the framework of FJI-H14 collapses when it is immersed for 24 h in solution at pH = 1 or pH = 13 (Supplementary Fig. 2 ). Thermogravimetric analysis (TGA) studies (Supplementary Fig. 3 ) indicate that the as-synthesized FJI-H14 sample is thermally stable up to 230 °C, and this is confirmed by temperature-dependent PXRD studies (Fig. 2b and Supplementary Fig. 4 ). Generally, MOFs based on Cu ions and organic carboxylates are usually subject to hydrolysis in the presence of moisture and only a few known MOFs show such excellent chemical stability [16] , [34] , [35] , [36] , [37] , [38] . The unusual chemical stability of FJI-H14 may result from its unique structure because the penta-coordinated Cu(II) ion subunit should be more stable than traditional paddle-wheel structure due to the Cu–N coordination interaction, which is stronger than the Cu–O interaction. Furthermore, the abundant free N atoms could also prevent the destruction caused by acids. Fig. 2 Stability of FJI-H14. a PXRD patterns after treatment with boiling water, acid/base environment from pH = 2 to 12 at 373 K. b Temperature-dependent PXRD patterns Full size image Porosity and CO 2 adsorption capacity The FJI-H14 sample for adsorption testing was pre-activated under dynamic vacuum at 100 °C for 10 h after exchanged by acetone for 3 days. PXRD data displayed that the crystallinity was retained after activation (Supplementary Fig. 5 ). N 2 adsorption at 77 K was much lower than expected (Supplementary Fig. 6 ), and consequently, the porosity of activated FJI-H14 was examined by CO 2 adsorption experiments at 195 K. A CO 2 uptake of 279 cm 3 g −1 was obtained (Fig. 3a ), corresponding to a formula [Cu(BTTA)] n ·4.5nCO 2 . 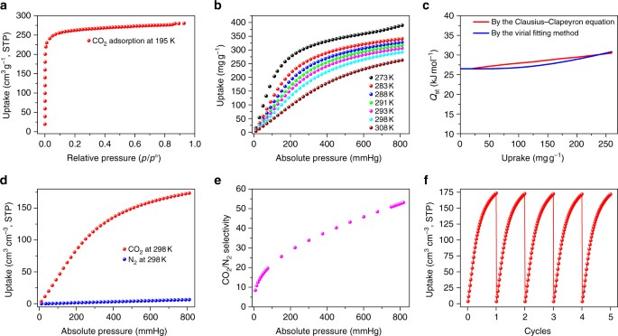Fig. 3 Experimental CO2adsorption by FJI-H14.aCO2adsorption isotherm forFJI-H14at 195 K.bCO2adsorption isotherm forFJI-H14at 273, 283, 288, 291, 293, 298 and 308 K.cThe isosteric heat of CO2adsorption (Qst) forFJI-H14calculated by the Clausius–Clapeyron equation and the Virial fitting method.dN2and CO2adsorption isotherms forFJI-H14at 298 K.eCO2/N2selectivity for the 15/85 CO2/N2mixture at 298 K.fCycles of CO2adsorption forFJI-H14at 298 K A phenomenon that restricted N 2 uptake at 77 K but supported type-I CO 2 uptake at 195 K has been observed in several reported MOF materials (Supplementary Table 3 ). However, FJI-H14 has a low N 2 uptake of 170 cm 3 g −1 at 77 K and 1 atm, which is different from the reported MOFs which exhibit almost zero N 2 adsorption at 77 K. The much lower N 2 adsorption at 77 K of FJI-H14 may be a consequence of the relatively narrow pores in FJI-H14 being easily blocked by the relatively large N 2 molecule at 77 K, so hindering further diffusion of N 2 into the framework of FJI-H14 . The typical type-I isotherm observed indicates that only micropores are formed in the framework of activated FJI-H14 . The Brunauer–Emmett–Teller (BET) -specific surface area of FJI-H14 is calculated to be 904 m 2 g −1 and its Langmuir-specific surface area is 1004 m 2 g −1 . The total pore volume estimated from the experimental CO 2 isotherm is 0.45 cm 3 g −1 at P/P 0 = 0.92, which is slightly higher than the theoretical value of 0.39 cm 3 g −1 derived from the solvent accessible volume and the crystal density through PLATON calculations with a probe radius of 1.65 Å. The comparable values of the pore volume indicate that the activated FJI-H14 remains permanently porous. Fig. 3 Experimental CO 2 adsorption by FJI-H14. a CO 2 adsorption isotherm for FJI-H14 at 195 K. b CO 2 adsorption isotherm for FJI-H14 at 273, 283, 288, 291, 293, 298 and 308 K. c The isosteric heat of CO 2 adsorption ( Q st ) for FJI-H14 calculated by the Clausius–Clapeyron equation and the Virial fitting method. d N 2 and CO 2 adsorption isotherms for FJI-H14 at 298 K. e CO 2 /N 2 selectivity for the 15/85 CO 2 /N 2 mixture at 298 K. f Cycles of CO 2 adsorption for FJI-H14 at 298 K Full size image The incorporation of high porosity and the high concentration of open active sites in the framework are expected to lead to high CO 2 uptake. Indeed, activated FJI-H14 exhibits remarkable CO 2 volumetric adsorption capacities of 171 cm 3 cm −3 at 298 K and 1 atm (Fig. 3d ), and the capacity is only lower than that of MAF-X25ox (203 cm 3 cm −3 ) [36] , MAF-X27ox (196 cm 3 cm −3 ) [36] and Co 2 (dobdc) (184 cm 3 cm −3 ) under the same conditions [36] , [39] , exceeding that in almost all well-known MOFs such as Mg-MOF-74 (162 cm 3 cm −3 ) [6] , [40] , UTSA-16 (160 cm 3 cm −3 ) [6] , [41] , SIFSIX-2-Cu-i (151 cm 3 cm −3 ) [42] , MPM-1-TIFSIX (115.7 cm 3 cm −3 ) [43] , Bio-MOF-11(113 cm 3 cm −3 ) [6] , [44] , Cu-tdpat(103 cm 3 cm −3 ) [6] , [45] and Mmen−CuBTTri (83 cm 3 cm −3 ) [6] , [30] (Supplementary Table 2 ). The formula of CO 2 adsorbed FJI-H14 at room temperature is [Cu(BTTA)] n ·2.4nCO 2 and there is a 53% CO 2 occupancy at room temperature compared with the maximal uptake at 195 K, which is rather high compared with reported MOFs such as SMT-1 (27%) [46] , [Cu(L)] (31%) [47] and MPM-1-Cl (29%) [43] . It should be noted that although volumetric adsorption capacity is more practical for stationary CO 2 capture and separation applications, the gravimetric adsorption capacity is also an important parameter for CO 2 capture. Although the gravimetric CO 2 uptake of FJI-H14 (146 cm 3 g −1 ) is lower than that of Mg-MOF-74 (176 cm 3 g −1 ) due to the considerably lighter weight of Mg [40] , it can be comparable to that in other familiar MOF materials such as MAF-X25ox (160 cm 3 g −1 ) [36] , [Co 2 (dobdc)] (154 cm 3 g −1 ) [39] or MAF-X27ox (150 cm 3 g −1 ) [36] . Another challenging issue is the uptake of CO 2 at low pressure, which can be highly improved by chemisorption due to the stronger interactions. For instance, the hydrazine functionalized MOF [Mg 2 (dobdc)(N 2 H 4 ) 1.8 ] (137 cm 3 cm −3 ) developed by Zhang et al. shows the highest volumetric CO 2 adsorption capacities at 298 K and 0.15 bar [31] , and the second highest is MAF-X27ox (124 cm 3 cm −3 ) [36] , which was also prepared by Zhang et al. Based on physisorption, FJI-H14 displays a volumetric capacity of 60 cm 3 cm −3 at 298 K and 0.15 atm, which makes it comparable to SIFSIX-2-Cu-i (63 cm 3 cm −3 ). In order to evaluate the affinity of the pore surface of activated FJI-H14 toward CO 2 , the isosteric heat of adsorption ( Q st ) of activated FJI-H14 was calculated using the Clausius–Clapeyron equation based on the CO 2 isotherms at seven different temperatures without data fitting (Fig. 3b , Supplementary Fig. 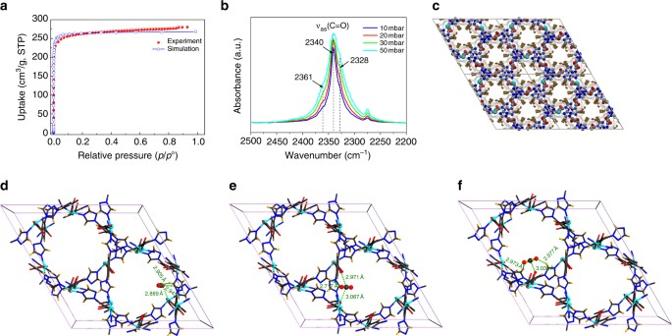Fig. 4 Mechanism of CO2adsorption of FJI-H14.aExperimental and simulated excess CO2adsorption isotherms at 195 K.bBackground-subtracted FTIR spectra of CO2adsorbed onFJI-H14at decreasing equilibrium pressure.cDensity picture of adsorbed CO2(1 CO2at 273 K), which is shown as a volume rendered mode.d–frepresent three preferential CO2locations inFJI-14obtained from GCMC simulation and DFT optimization 7 and Supplementary Table 4 ). As shown in Fig. 3c , the Q st at low coverage is 26.6 kJ mol −1 and then slightly increases to 30.5 kJ mol −1 with CO 2 loading increasing to 260 mg g −1 . The Q st with an increasing slope is unusual [9] , [36] , [43] , [48] , and reveals the possible formation of CO 2 clusters inside the pores. Such phenomena have been previously observed in other porous MOFs materials [41] , [49] . The Q st , confirmed by the Virial fitting method [50] , also slowly increases from 26.5 to 30.8 kJ mol −1 with increasing CO 2 loading from lower coverage to 260 mg g −1 (Fig. 3c and Supplementary Fig. 8 ). Such similar trends in the two methods confirm the unusual increasing slope in Q st . Because flue gas from power plants contains a large amount of N 2 , the CO 2 /N 2 selectivity is a crucial parameter in CO 2 capture applications. For comparison, N 2 sorption isotherms were also measured at 298 K, and showed an uptake of 6.5 cm 3 cm −3 at 1 atm (Fig. 3d ). By the ideal adsorbed solution theory (IAST) [51] , the CO 2 /N 2 selectivity for the 15/85 CO 2 /N 2 mixture at 1 atm is calculated to be 51 at 298 K (Fig. 3e ). The highly selective adsorption of CO 2 over N 2 further suggests that the densely populated open active sites in the framework have a positive effect on CO 2 adsorption. The possibility of reuse of an adsorbent is also an important aspect of the practical application. Further research demonstrates that activated FJI-H14 can be recycled without losing its adsorption capacity. Even after five cycles, it still maintains 100% adsorption capacity as shown in Fig. 3f , indicating that FJI-H14 is highly suitable for CO 2 capture. Revealing the CO 2 adsorption sites in FJI-H14 The extraordinary CO 2 capture performance of FJI-H14 under ambient conditions has motivated us to rationalize the crucial factors supporting the high CO 2 adsorption capacity. To understand the sorption behavior of FJI-H14 , both grand canonical Monte Carlo (GCMC) simulations and density functional theory (DFT) calculations have been carried out and are shown in Fig. 4 . The GCMC simulations show that the theoretical CO 2 adsorption isotherms of FJI-H14 are basically consistent with the experimental data at different temperatures (195, 273 and 298 K) (Fig. 4a , Supplementary Fig. 9 ). The simulated CO 2 concentration loaded into FJI-H14 is about 4.3, 3.1 and 2.5 CO 2 per ligand molecule at 195, 273 and 298 K, respectively. These figures are close to the experimental values of 4.5, 3.1 and 2.4 CO 2 per ligand molecule at 195, 273 and 298 K. As shown in Fig. 4c , the adsorbed CO 2 molecules at low coverage prefer to locate the corners of hexagonal channels. Combining the density plots and a snapshot of the adsorbed CO 2 molecules, three typical preferential CO 2 adsorption sites can be observed. These three adsorption sites were further optimized by DFT methods using the Dmol [3] module. Site I (Fig. 4d ) shows that CO 2 molecules prefer to coordinate with open Cu(II) ions through Cu–O interaction, with a Cu–O distance of about 2.889 Å, and each copper site binding only one CO 2 [52] . In Site II (Fig. 4e ), the two closest C–O distances are about 2.971 and 3.067 Å, indicating that O atoms of carboxyl group could also interact as a Lewis base with CO 2 . It is also interesting to find that positively charged H atoms could further promote CO 2 adsorption, with the shortest O-H distances about 2.577 Å as shown in Site III (Fig. 4f ). The calculated static CO 2 binding energy of the above three different preferential CO 2 adsorption sites are ~43.71, 38.94, 32.82 kJ mol −1 , respectively, indicating that the open copper sites could play a leading role in CO 2 adsorption. Fig. 4 Mechanism of CO 2 adsorption of FJI-H14. a Experimental and simulated excess CO 2 adsorption isotherms at 195 K. b Background-subtracted FTIR spectra of CO 2 adsorbed on FJI-H14 at decreasing equilibrium pressure. c Density picture of adsorbed CO 2 (1 CO 2 at 273 K), which is shown as a volume rendered mode. d – f represent three preferential CO 2 locations in FJI-14 obtained from GCMC simulation and DFT optimization Full size image The simulated Q st from the GCMC simulations can be used to deduce the information on Q st with an increasing slope for FJI-H14 . As shown in Supplementary Fig. 10 , the simulated Q st of 30.7–34.6 kJ mol −1 is slightly larger than suggested by experimental results and has a uniformly increasing trend with increasing CO 2 loading. The contribution of the CO 2 ···Framework interaction to the total Q st decreases slightly with increasing loading, which is reasonable because CO 2 molecules first occupied the more active sites. However, the contribution from the CO 2 ···CO 2 interactions shows a tendency to increase significantly from 0 to 7.0 kJ mol −1 , which is due to the closer packing of the CO 2 molecules under the higher pressure in the relatively narrow pores. Hence, the behavior of the total Q st is the result of the two cooperative contributions. The increasing contribution from the CO 2 ···CO 2 interactions indicates that the CO 2 clusters could have formed inside the pores. Hence, GCMC simulation was used to investigate the potential CO 2 clusters. Some small CO 2 clusters can be found in the snapshot at 195 K and low pressure (~ 21 Pa) calculated using the GCMC method (Supplementary Fig. 11 ), but at 273 K, similar CO 2 clusters can only be observed under a relatively high pressure of 11 kPa. The snapshots of the framework of FJI-H14 with CO 2 molecules adsorbed are shown in Fig. 5a . The weak interactions between neighboring CO 2 molecules are found in terms of the short C···O separation (from 2.71 to 3.50 Å) for adjacent CO 2 molecules, which links those CO 2 molecules into small clusters (Fig. 5b and Supplementary Fig. 12 ). Fig. 5 The snapshot for CO 2 -loaded FJI-H14. a The snapshot of CO 2 adsorption for FJI-H14 at 11.2 kPa and 273.15 K calculated using the GCMC method. b The representative CO 2 clusters including nine (C9), six (C6), five (C5) and four (C4) CO 2 molecules. The blue dashed line represents weak interactions between neighboring CO 2 molecules with a short C···O separation (from 2.71 to 3.50 Å) for adjacent CO 2 molecules Full size image To verify the preferential adsorption sites experimentally, in situ fourier transform infrared microscope (FT-IR) spectra of activated FJI-H14 sample have been collected at increasing equilibrium pressure under a CO 2 atmosphere. Figure 4b shows the background-subtracted IR spectra obtained by the progressive lowering of equilibrium pressure at room temperature. The strong absorption bands at 2,340 and 2,328 cm −1 red-shifted by Δ ν of about −9 and −21 cm −1 from gas phase CO 2 asymmetric stretch ( ν as = 2349 cm −1 ) might be attributed to the ν as mode of CO 2 (Supplementary Fig. 13 ) interacting with Cu(II) centers. The slightly blue-shifted band at 2,361 cm −1 (Δ ν =  + 12 cm −1 shift) can be readily assigned to the asymmetric ν as stretch of CO 2 interacting with the exposed Lewis base sites throughout the channel. On the low-frequency side of this main absorption, the less intense bands at 2,275 cm −1 result from the interaction between Cu(II) center and 13 CO 2 which is present (1%) naturally in 12 CO 2 . The stronger absorption bands at 2,340 cm −1 and 2,328 cm −1 also indicate that CO 2 molecules tend to stack around the open Cu(II) sites, which is in accord with the above theoretical calculation. Large-scale synthesis For practical applications, efficient macroscopic preparation and purification are a bottleneck problem which must be solved. After many attempts, the following protocol for large-scale preparation of FJI-H14 has been established: by directly mixing H 2 BTTA ligand and Cu(NO 3 ) 2 in water and then refluxing for 1 day, microcrystalline FJI-H14 can be obtained with a high yield of 90%, its purity confirmed by PXRD analysis (Fig. 6b ). Scanning electron microscopy measurements demonstrate that the relatively uniform rod crystallites form on the scale of about 20 μm, displaying a similar morphology with the single crystal (Fig. 6a ) obtained from the hydrothermal reaction. Therefore, macroscopic samples of FJI-H14 even on a 10 g scale can be readily synthesized by this method, which makes its application more possible. Fig. 6 Large-scale synthesis of FJI-H14 microcrystals. a Morphology comparison between SEM image of FJI-H14 microcrystals and of FJI-H14 single crystals (inset). Scale bars, 10 µm. b PXRD patterns comparison: black represents simulated FJI-H14 ; red represents FJI-H14 microcrystals Full size image Catalyzed cycloaddition of CO 2 using flue gas as feedstock Another attractive means of effective elimination of CO 2 is the direct chemical conversion of CO 2 into value-added chemicals, such as dimethyl carbonate, cyclic carbonates, N , N ’-disubstituted ureas or formic acid. Given their wide applications in the pharmaceutical and fine chemical industries, cyclic carbonates formed by the coupling of epoxides with CO 2 have attracted intense interest. Although several existing MOFs have been shown to be excellent heterogeneous Lewis acid catalysts for chemical conversion of CO 2 either at high pressure or normal pressure [53] , [54] , [55] , [56] , the exploration of practically useful MOF materials which can catalyze the conversion of CO 2 obtained directly from power plants remains a challenge to be addressed. The high density of OMSs and LBSs which are finely distributed throughout the channel pores of FJI-H14 , are devoted to capturing CO 2 effectively and selectively under ambient conditions. Such unusual synergistic effects may also improve chemical conversion of post-combustion CO 2 from the power plant. Here, we use a mixed gas which contains 0.15 atm CO 2 and 0.85 atm N 2 to simulate flue gas from the power plant. As expected, FJI-H14 displays a much higher catalytic activity for cycloaddition of styrene oxide with the simulated flue gas than other catalysts, such as homogeneous Cu(OAc) 2 , heterogeneous HKUST-1 and a mixture of Cu(NO 3 ) 2 and free H 2 BTTA ligand. As shown in Table 1 , absence of extra Lewis acid catalysts only lead to a moderate yield (52%), while use of extra Cu(II) catalyst can improve their reaction activity, with the exception of Cu(OAc) 2 . Catalyzed by FJI-H14 , chemical conversion of diluted CO 2 with styrene oxide into corresponding cyclic carbonates gives a yield of 86% within 24 h, while use of homogeneous Cu(OAc) 2 and the mixture of Cu(NO 3 ) 2 and H 2 BTTA leads only to 45 and 70% yields respectively under the same reaction conditions. Further tests demonstrate that the FJI-H14 is more active than well-known HKUST-1 which leads to only 67% yield under the same conditions. All these results indicate that FJI-H14 is indeed an efficient catalyst for chemical conversion of CO 2 under practical conditions. In order to investigate the catalytic character of FJIH-14 , another two different sized substrates have been selected. As shown in Table 1 entries 5–6, the smaller (chloromethyl)ethylene oxide gives a higher yield (95%), while 1,2-epoxyoctane leads to a lower yield (27%), indicating that the cycloaddition reaction may occur within the pores of FIJ-H14 , into which smaller-sized substrates could easily diffuse and make contact with the active sites. To further prove that the reaction may occur in the pores of FJI-H14 , uptake of different reactants has also been assessed. Further analysis demonstrates that (chloromethyl)ethylene oxide indeed diffuses into the pores of FJI-H14 more easily than 1,2-epoxyoctane and styrene oxide which apparently have similar diffusion rates. Considering the similar diffusion from 1,2-epoxyoctane and styrene oxide, the higher activity of styrene oxide compared to 1,2-epoxyoctane may result from following two factors: first, a phenyl ring is an electron-withdrawing group, which can improve reaction activity, and second, the π–π interaction from the phenyl ring of styrene oxide and the aromatic rings of the FJI-H14 framework also can improve reaction activity. This may provide a strategy for development of more practical catalysts for the conversion of CO 2 directly from flue gas. Table 1 Cyclic carbonates from epoxides and CO 2 a Full size table Considering that most of CO 2 emission is generated from power stations, direct elimination of such CO 2 should play an important role in the reduction of global CO 2 emissions. The characteristics and composition of post-combustion CO 2 determine that an ideal adsorbent for post-combustion CO 2 capture should possess advantages such as high CO 2 uptake and selectivity at ambient pressure, excellent chemical stability and thermal stability, good reusability and large-scale production with low cost. Porous MOFs have been proved to be effective adsorbents for CO 2 capture due to their large capacity for the adsorption of gases, but development of an ideal MOF for post-combustion CO 2 capture is still challenging. Although many different OMS and LBS have been introduced into MOFs to improve CO 2 capture, only very few porous MOFs have been realized for high CO 2 capture at ambient conditions, and most of them are sensitive to water. FJI-H14 not only shows extraordinary high volumetric uptake of CO 2 with high selectivity under ambient conditions but is also highly resistant to water and an acid/base environment; furthermore, it also can be reused without loss of adsorption capacity and prepared on a large-scale with low cost. These advantages make FJI-H14 an ideal and practical adsorbent for post-combustion CO 2 . An unusual synergistic effect from multiple active sites has also been observed, and may provide a strategy for the design of more effective adsorbents for CO 2 capture. Further chemical conversion of captured CO 2 to high-value products, such as cyclic carbonate, is also attractive, and several existing MOFs have been proved to be excellent heterogeneous Lewis acid catalysts for chemical conversion of pure CO 2 . However, development of MOF materials which can catalyze the direct conversion of post-combustion CO 2 still remains a challenge. It is shown here that FJI-H14 can directly and smoothly catalyze the chemical transformation of simulated post-combustion gas CO 2 into corresponding cyclic carbonates. All these results should be instructive for the design and discovery of more effective and practical MOF materials for the elimination of post-combustion CO 2 in the near future. Synthesis and scale up A mixture of Cu(NO 3 ) 2 ·3H 2 O (0.05 mmol, 12 mg) and H 2 BTTA (0.05 mmol, 15 mg) in H 2 O (4 ml) was sealed in a 23 mL Teflon vial, which was heated at 120 °C for 3 days, then cooled to room temperature. After washing with fresh acetone, blue crystals of FJI-H14 were obtained in 73% yield based on the organic ligand H 2 BTTA. Elemental analysis was calculated for FJI-H14 : C, 29.54%; H, 4.13%; N, 17.23%. Found: C, 29.35%; H, 4.12%; N, 17.29%. For scale up, a mixture of Cu(NO 3 ) 2 ·3H 2 O (1 mmol, 241.6 mg) and H 2 BTTA (1 mmol, 300.1 mg) in H 2 O (80 ml) was refluxed for 1 day, and then the blue powder of FJI-H14 microcrystals could be obtained in 90% yield based on H 2 BTTA. After three washings with water and two with acetone, the phase purity of the sample was confirmed by PXRD. Characterization Elemental analyses for C, H, N were carried out on a German Elementary Vario EL III instrument. The 1 H NMR spectra were measured on an AVANCE III Bruker Biospin spectrometer, operating at 400 MHz. Thermogravimetric analyses (TGA) were recorded on an NETZSCH STA 449 C unit at a heating rate of 10 °C min −1 under flowing nitrogen atmosphere. In situ FT-IR spectra were obtained using a NICOLET 6700 instrument at 298 K. The PXRD patterns were collected using a Rigaku MiniFlex 600 X-ray diffractometer with monochromatic Cu Kα radiation ( λ = 1.54 Å). Simulations of the PXRD spectrum were carried out by the single-crystal data and diffraction-crystal module of the Mercury program, available free of charge via the internet at https://www.ccdc.cam.ac.uk/solutions/csd-system/components/mercury/ . Single-crystal X-ray diffraction The single-crystal data of FJI-H14 was collected on a SuperNova diffractometer at 100 K. The structure was solved using SHELXT -2014 and refined by full-matrix least squares on F 2 with SHELXL -2014 [57] . All the non-hydrogen atoms were refined anisotropically. Hydrogen atoms of the organic ligands were generated theoretically onto the specific atoms and refined isotropically. We employed PLATON/SQUEEZE [58] to calculate the contribution to the diffraction from the solvent region and thereby produced a set of solvent-free diffraction intensities. The final formula was calculated from the SQUEEZE results combined with elemental analysis data and TGA data. Crystallographic data and structure refinement parameters for this crystal are summarized in Supplementary Table 1 . Gas-adsorption Low-pressure (<1 bar) adsorption measurements were performed using an Accelerated Surface Area and Porosimetry 2020-M System. Before the measurements, about 100 mg solvent-exchanged samples were loaded into the sample tube and then degassed under dynamic vacuum at 100 °C for 10 h to obtain fully desolvated samples. Low-pressure N 2 adsorption isotherms were measured at 77 K in a liquid nitrogen bath (Supplementary Fig. 6 ). Low-pressure CO 2 adsorption isotherms were measured at 195, 273, 283, 288, 291, 293, 298 and 308 K. The specific surface areas were determined using the BET model from the CO 2 adsorption isotherm. The isosteric heat of adsorption Method 1: the isosteric heat of adsorption Q st was calculated using the Clausius–Clapeyron equation (equation ( 1 )). ln( P_i) = Q_st×1/RT_i + C,
 (1) where P i is the pressure of the isotherm i (kPa), T i is the temperature of isotherm i (K), R is the gas constant and C is a constant. The Qst is subsequently obtained from the slope of plots of ln( P i ) as a function of 1/T (Supplementary Fig. 7 and Supplementary Table 4 ). Method 2: the Qst was estimated from isotherms at different temperatures applying the Virial fitting method (equation ( 2 ) and Supplementary Fig. 8 ). The fitting parameters were then used to calculate the Q st using equation ( 3 ). ln P = ln N + 1/T∑_i = 0^m a_iN^i + ∑_i = 0^n b_iN^i ,
 (2) 
    Q_st = - R∑_i = 0^m a_iN^i ,
 (3) where P is the pressure (mmHg), N is the adsorbed quantity (mg g −1 ), T is the temperature (K), R is the gas constant, a i and b i are virial coefficients and m and n represent the number of coefficients required to adequately describe the isotherms (herein, m = 5, n = 2). Calculation of gas selectivity based on IAST The gas adsorption isotherms were first fitted to a Langmuir-Freundlich model. IAST starts from the Raoults’ Law type of relationship between fluid and adsorbed phase. P_i = Py_i = P_i^ox_i,
 (4) 
    ∑_i = 1^n x_i = ∑_i = 1^n P_i/P_i^0 = 1,
 (5) where P i is the partial pressure of component i (kPa), P is the total pressure (kPa), y i and x i represent mole fractions of component i in gas and adsorbed phase (dimensionless). \(P_i^0\) is the equilibrium vapor pressure (kPa). In IAST, \(P_i^0\) is defined by relating to spreading pressure π, 
    π S/RT = ∫_0^P_i^0q_i(P_i)/P_idP_i = Π ( Constant),
 (6) where π is the spreading pressure, S is the specific surface area of adsorbent (m 2 g −1 ), R is the gas constant, T is the temperature (K) and q i ( P i ) is the single component equilibrium obtained from the isotherm (mg g −1 ). The isotherm parameters are known from the previous fitting. The adsorption selectivities S ads were calculated using equation ( 7 ). S_ads = q_1/q_2/p_1/p_2. (7) In this study, IAST calculations were carried out assuming CO 2 /N 2 (15/85) binary mixed gases at 298 K and pressure up to 1 bar to mimic the composition and condition of flue gas for post-combustion CO 2 capture. Computational methodologies The GCMC simulations for CO 2 at 195, 273 and 298 K and up to 100 kPa were performed using with RASPA v2.03 [59] . The FJI-H14s framework was generated in the R 3 space group based on the crystallographic data of FJI-H14 to avoid disorder in the structure (Supplementary Fig. 14 ). Twelve unit cells of FJI-H14s (2 × 2 × 3) were used to construct the simulation box of the GCMC run. The structural parameters of simulation box are a = b = 44.9714 Å and c = 33.1527 Å, as well as α = β = 90° and γ = 120°. The partial charges on the framework atoms were calculated by the Gaussian09 software at the B3LYP/6–31 G* level of theory [60] . Partial atomic charges were extracted using the ChelpG method by fitting them to reproduce the electrostatic potential generated by the DFT calculations. The charge was adjusted slightly in order to result in a neutral framework. 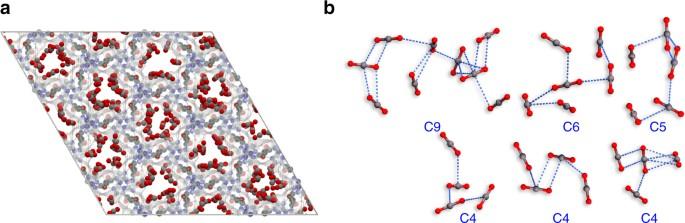Fig. 5 The snapshot for CO2-loaded FJI-H14.aThe snapshot of CO2adsorption forFJI-H14at 11.2 kPa and 273.15 K calculated using the GCMC method.bThe representative CO2clusters including nine (C9), six (C6), five (C5) and four (C4) CO2molecules. The blue dashed line represents weak interactions between neighboring CO2molecules with a short C···O separation (from 2.71 to 3.50 Å) for adjacent CO2molecules Resulting partial charges for FJI-H14s are given in Supplementary Table 5 . CO 2 –CO 2 and CO 2 -framework interactions were calculated using a Lennard–Jones (LJ) + Coulomb potential. LJ parameters for the framework atoms were taken from the Dreiding Force Field except for the copper atom, for which the parameters were taken from UFF (Supplementary Table 7 ). 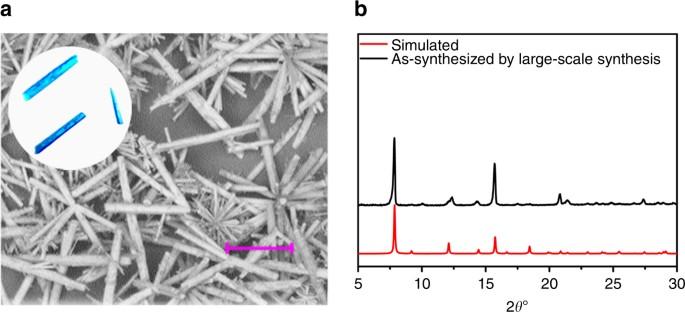Fig. 6 Large-scale synthesis of FJI-H14 microcrystals.aMorphology comparison between SEM image ofFJI-H14microcrystals and ofFJI-H14single crystals (inset). Scale bars, 10 µm.bPXRD patterns comparison: black represents simulatedFJI-H14; red representsFJI-H14microcrystals The CO 2 LJ parameters were taken from an empirical TraPPE force field with a partial charge on each atom (Supplementary Table 6 ). The mixing LJ parameters between different atomic types were calculated according to the Lorentz–Berthelot mixing rule. Lorentz–Berthelot mixing rules were used for all cross terms, and LJ interactions beyond 12.8 Å were neglected. The Ewald sum method was used to compute the electrostatic interactions. The fugacity of CO 2 was calculated using the Peng-Robinson equation of state with the corresponding parameters. Simulations for CO 2 adsorption used 100,000 cycles for equilibration and 100,000 cycles for data collection. In a cycle, N Monte Carlo moves were performed, where N is whichever value is larger between 20 and the number of molecules in the system. Monte Carlo moves used with equal probability were translation, rotation, insertion, deletion, and random reinsertion of an existing molecule at a new position, while framework atoms remained fixed at their original positions. The simulated isosteric heats of adsorption are computed from the GCMC simulations using the expression (equation ( 8 )). Q_st = RT - ⟨U_ggN⟩ - ⟨ U_gg⟩⟨ N⟩/⟨N^2⟩ - ⟨ N ⟩ ^2 - ⟨ U_gfN⟩ - ⟨ U_gf⟩⟨ N⟩/⟨ N^2⟩ - ⟨ N⟩^2,
 (8) where the brackets 〈 〉 denote the ensemble average, R is the gas constant, N is the number of gas molecules in the system, U gg is gas···gas interaction energy and U gh is the gas···framework interaction energy. The second and third terms are the contributions to the simulated Q st from the gas···gas interaction and the gas···framework interaction, respectively. DFT methods help shed light on adsorption mechanisms by calculating the adsorption energy of CO 2 in MOF. Three possible main adsorption sites for adsorbed CO 2 in MOF were investigated by the Dmol [3] module integrated into the Material Studio 7.0 program package [61] . The PBE-type exchange-correlation functional [62] with a generalized gradient approximation and the Double Numerical plus polarization (DNP) basis sets [63] that include a d-type polarization function on all non-hydrogen atoms and a p-type polarization function on all hydrogen atoms were employed for all calculations [64] . The FINE quality mesh size was employed in the calculations. During the CO 2 -MOF structure optimization, the lattice parameters and the atomic fraction positions of the MOF crystal were kept immobile and the single CO 2 molecule was allowed to move during optimization. The possible adsorption sites are shown in the Fig. 4d–f . The adsorption energies were calculated in terms of equation ( 9 ) 
    E_ads = E_MOF - CO_2 - E_MOF - E_CO_2,
 (9) where \({E_{{\rm{MOF}} - {\rm{C}}{{\rm{O}}_2}}}\) stands for the energy of the optimized adsorbate-MOF structure, and E MOF , and E CO2 denote the energies of the bare MOF structure and the isolated CO 2 molecule, respectively. According to this equation, a more negative adsorption energy means more favorable binding. Catalyzation of cycloaddition of simulated post-combustion CO 2 20 mmol styrene oxide, 0.48 mol% per Cu(II) units (for example, 18 mg activated FJI-H14 (0.016 mmol), 8.7 mg Cu(OAc) 2 (0.048 mmol)), and 164 mg TBAB (0.5 mmol, 2.5 mol%) were placed in a 5 mL dry Schleck tube with condenser, then 1 atm simulated post-combustion flue gas (CO 2 = 0.15 atm, N 2 = 0.85 atm) was introduced by bubbling, and the reaction mixture was stirred at 80 °C for 24 h. Uptake of different reactants 10 mg of activated crystals of FJI-H14 was placed in a dry 5 ml Schleck flask, the flask was then evacuated under dynamic vacuum at 80 °C for 2 h and filled with argon, then 1 ml reactant was injected and the reaction was kept under argon atmosphere. 10 min later, the inclusion crystals of FJI-H14 were filtered, after removing surface reactant molecules; the inclusion reactants can be readily removed from inclusion crystals FJI-H14 by ultrasonic processing in DMSO-d 6 solution and further determined by 1 H NMR. Finally, about 2.78 μmol of (chloromethyl)ethylene oxide, 1.2 μmol of 1,2-epoxyoctane, or 1.1 μmol of styrene oxide were added. Data availability The X-ray crystallographic coordinates for structure reported in this article have been deposited at the Cambridge Crystallographic Data Centre (CCDC), under deposition number CCDC 1517725. These data can be obtained free of charge from The Cambridge Crystallographic Data Centre via www.ccdc.cam.ac.uk/data_request/cif .